Nucleosomal occupancy changes locally over key regulatory regions during cell differentiation and reprogramming Chromatin structure determines DNA accessibility. We compare nucleosome occupancy in mouse and human embryonic stem cells (ESCs), induced-pluripotent stem cells (iPSCs) and differentiated cell types using MNase-seq. To address variability inherent in this technique, we developed a bioinformatic approach to identify regions of difference (RoD) in nucleosome occupancy between pluripotent and somatic cells. Surprisingly, most chromatin remains unchanged; a majority of rearrangements appear to affect a single nucleosome. RoDs are enriched at genes and regulatory elements, including enhancers associated with pluripotency and differentiation. RoDs co-localize with binding sites of key developmental regulators, including the reprogramming factors Klf4, Oct4/Sox2 and c-Myc. Nucleosomal landscapes in ESC enhancers are extensively altered, exhibiting lower nucleosome occupancy in pluripotent cells than in somatic cells. Most changes are reset during reprogramming. We conclude that changes in nucleosome occupancy are a hallmark of cell differentiation and reprogramming and likely identify regulatory regions essential for these processes. Embryonic stem cells (ESCs) and induced-pluripotent stem cells (iPSCs) self-renew and differentiate into various cell types in vitro and in vivo . A complex network of genetic and epigenetic pathways regulates their self-renewal and differentiation, and the structural organization of chromatin play a prominent role in these processes. Prior studies have established multiple unique properties of pluripotent chromatin and its regulation, including macrostructural descriptions of ESC chromatin as relatively ‘open’ compared with lineage-committed cells [1] , [2] , [3] , [4] , [5] , [6] . The pluripotency factors Oct4, Sox2 and Nanog transcriptionally regulate and interact with specific chromatin-remodeling and histone-modifying complexes [7] . Reciprocally, multiple chromatin regulators, including complexes unique to ESCs, have been implicated in the maintenance of pluripotency, cellular differentiation and development [1] , [2] , [3] , [8] , [9] , [10] . The physical packaging of DNA into nucleosomes is a central determinant of DNA accessibility in both cis and trans . Nucleosomes consist of ~150 bp of DNA wrapped around a core histone octamer [11] , [12] . Nucleosome positioning on genomic DNA is dynamic and influences regulatory factor binding, which impacts processes ranging from gene regulation to DNA replication, recombination and repair [13] , [14] . Thus, characterizing changes in nucleosome occupancy should reveal important regulatory features in pluripotent cell biology, differentiation and reprogramming. Information on nucleosome location can be integrated with previous studies on covalent changes to chromatin (for example, DNA and histone methylation, histone acetylation) to improve our understanding of how chromatin dynamics contribute to pluripotency. Techniques that map nucleosome positioning on the genome scale have illuminated the role of primary chromatin structure in the mammalian cell [15] , [16] , [17] , [18] , [19] , [20] , [21] , [22] . However, comparing the nucleosome profiles between different cell types still presents profound challenges. Observed nucleosome occupancy is sensitive to even slight variations in experimental conditions, such as the degree of chromatin fragmentation or chromatin isolation conditions [23] , [24] . This variability is hard to control and, as a result, changes in nucleosome occupancy and positioning associated with biological processes in mammals have been difficult to quantify. In particular, it is not clear if large-scale or local nucleosome profile rearrangements are prevalent upon cell fate change—how these rearrangements contribute to alterations in gene expression, and if nucleosome profiles are reset completely upon cell reprogramming. Here we investigate nucleosome occupancy within pluripotent and somatic cells and identify regions of differences (RoD) between ESCs, iPSCs and somatic cells in both mouse and human. This analysis is facilitated by a novel data processing method developed for pairwise comparisons of nucleosome occupancy measured in different conditions and cell types. We report that the observed differences mostly do not appear to exceed the size of single nucleosomes, are enriched for motifs of transcription factors (TFs) that drive pluripotency and somatic cell reprogramming, and reside within gene regulatory regions, specifically at transcriptional start sites (TSSs) and enhancers of genes linked to pluripotency and differentiation. These findings reveal that localized changes in nucleosome occupancy at key regulatory regions, rather than large-scale rearrangements, may be sufficient to impact cell identity. Nucleosome mapping in pluripotent and somatic cells The results of this study are primarily based on the analysis of primary chromatin structure in three murine cell types: mouse ESCs, iPSCs derived from tail-tip-fibroblasts (iPSC-TTFs) and somatic TTFs. We also used somatic liver cells for validation purposes. All cells originated from the same isogenic mouse line and were previously characterized [25] . For each cell type, we created a genome-wide profile of nucleosome occupancy. To this end, we measured DNA protection patterns after chromatin digestion by micrococcal nuclease (MNase), building upon strategies previously developed by our group and others [15] , [17] , [20] , [26] , [27] , [28] , [29] . MNase selectively cleaves chromatin in linker DNA between nucleosomes, allowing a detailed description of nucleosome occupancy in a given cell population. The digestion fragments were size-selected and subjected to high-throughput sequencing, generating over 100 million mapped paired-end reads for each cell type. The average fragment size for each library was near the predicted mononucleosomal DNA length (~150 bp), and libraries showed high complexity with low percentages of repeats. We note that while the majority of the sequenced fragments likely represent nucleosome-associated DNA, some fragments may originate from loci protected by non-histone proteins, such as TFs [30] . Conversely, due to the preferential elimination of longer fragments during library preparation and sequencing, our data set may be depleted of the nucleosomes bound by larger complexes such as Pol II [31] . With these limitations in mind, we use the term nucleosome occupancy to characterize the number of digestion fragments at a given genomic position. For comparison and validation of our results, we also used human ESCs, fibroblast-derived human iPSCs and differentiated fibroblasts (referred here as hESCs, hiPSCs and human fibroblasts, respectively). Here we emphasize the data from mouse cells, as we have a greater number of isogenic cell types for comparison and these data displayed higher reproducibility in our analyses. Importantly, the same trends were observed in the data derived from human samples (for more details, see Supplementary Material ). We first assessed the average nucleosome occupancy patterns at the TSSs for each cell type. As demonstrated previously [16] , [17] , [19] , [26] , a nucleosome depleted region (NDR) flanked by well-positioned +1 and −1 nucleosomes (relative to the TSS) is a characteristic feature of the occupancy profiles averaged across all genes ( Fig. 1 ). Indeed, we detected such a pattern across all samples ( Fig. 1a ). However, we also observed high variability in the magnitude of the nucleosome occupancy for ESCs and iPSCs, which show nearly identical gene expression patterns in both the mouse and human data ( Fig. 1a and Supplementary Figs 1 and 4 ). Furthermore, such variation was observed even for biological replicates of the same cell type. This variability is not specific to our experimental protocol, as previous studies in mammalian genomes reported substantially different nucleosomal patterns at TSSs, ranging from an accumulation in tag counts greater than the surrounding regions to an apparent depletion in occupancy [16] , [17] , [18] , [19] , [22] , [32] . Thus, it likely originates from technical differences in experimental procedures, such as the extent of MNase digestion or chromatin isolation. This variability hinders direct comparisons of the nucleosome occupancy between cell types. 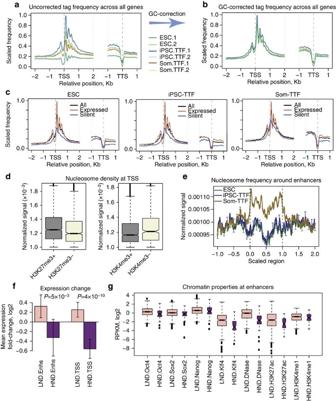Figure 1: Comparison of nucleosome occupancy in mouse pluripotent and somatic cells. (a) Nucleosome occupancy around transcription start and end sites computed for mouse ESCs, iPSCs and somatic TTFs. We note that after normalizing the occupancy for the total number of tags in each library the profiles remain different, even between replicates of the same cell type. (b) The same profiles after normalization of the GC-content distribution in each sample with the target mean GC content of 50% (see Methods for more detail). (c) Comparison of the GC-normalized profiles for all genes and genes stratified by their expression status. (d) Boxplots showing nucleosome density distributions in TSS-proximal regions (±2 kb) stratified by the enrichment in H3K4me3 and K3K27me3 marks in ESCs. Notches at boxes provide reference to 95% confidence intervals. (e) Normalized nucleosome occupancy signal around scaled ESC enhancer regions computed for replicate sets in three cell types. Vertical arrows represent standard errors of mean. (f) Comparison of gene expression and nucleosome occupancy changes. The two left bars show the expression changes computed for genes assigned to enhancers that have either lower (LND, pink) or higher (HND, purple) nucleosome occupancy in ESCs as compared with somatic TTFs; the two right bars depict the same for genes where nucleosome occupancy loss or gain occurs in the TSS-proximal regions. The 95% confidence intervals are shown with vertical arrows. (g) Comparison of the different chromatin properties (measured in ESCs40) for the LND and HND enhancers. As ind, notches provide 95% confidence intervals. Figure 1: Comparison of nucleosome occupancy in mouse pluripotent and somatic cells. ( a ) Nucleosome occupancy around transcription start and end sites computed for mouse ESCs, iPSCs and somatic TTFs. We note that after normalizing the occupancy for the total number of tags in each library the profiles remain different, even between replicates of the same cell type. ( b ) The same profiles after normalization of the GC-content distribution in each sample with the target mean GC content of 50% (see Methods for more detail). ( c ) Comparison of the GC-normalized profiles for all genes and genes stratified by their expression status. ( d ) Boxplots showing nucleosome density distributions in TSS-proximal regions (±2 kb) stratified by the enrichment in H3K4me3 and K3K27me3 marks in ESCs. Notches at boxes provide reference to 95% confidence intervals. ( e ) Normalized nucleosome occupancy signal around scaled ESC enhancer regions computed for replicate sets in three cell types. Vertical arrows represent standard errors of mean. ( f ) Comparison of gene expression and nucleosome occupancy changes. The two left bars show the expression changes computed for genes assigned to enhancers that have either lower (LND, pink) or higher (HND, purple) nucleosome occupancy in ESCs as compared with somatic TTFs; the two right bars depict the same for genes where nucleosome occupancy loss or gain occurs in the TSS-proximal regions. The 95% confidence intervals are shown with vertical arrows. ( g ) Comparison of the different chromatin properties (measured in ESCs [40] ) for the LND and HND enhancers. As in d , notches provide 95% confidence intervals. Full size image Among the characteristics of MNase-seq data that correlate with the degree of MNase digestion is the GC-content distribution of the sequenced fragments, which noticeably varied across all samples including biological replicates ( Supplementary Fig. 2 ). The GC content of a population of MNase-digested DNA fragments can change with increasing or decreasing digestion levels [33] . This is in part due to MNase bias towards cutting AT-rich sequences, and in part due to preferential digestion of genomic regions with different accessibility and base composition. We expected GC-content distribution to be similar between replicates given our careful control of digestion conditions, DNA fragment selection and library preparation; however, we still observed variability. To address this issue, we implemented a step in our methodology that used the GC content of DNA sequence as a metric for normalization. Previously, nucleotide composition, including GC-content normalization, has been applied to the analysis of microarray and high-throughput sequencing data [34] , [35] , [36] . Here we applied a concept used for ChIP-seq data [35] to the data produced by MNase digestion assays ( Supplementary Fig. 3 ). We normalized GC content in each sample to 50%, which roughly corresponds to the average GC content in the TSS-proximal regions in the genome. The GC-content normalization markedly reduced variability across all TSS-proximal profiles in both murine and human data ( Fig. 1a,b and Supplementary Fig. 4A,B ). Since TSS-proximal profiles are produced by averaging across large sets of genomic loci, they should be similar for samples demonstrating similar gene expression patterns, especially for replicates of the same cell type. To evaluate the extent of similarity, we computed correlation between nucleosome densities at TSSs in different samples (measured as average normalized frequency of fragments per kilobase of DNA) and observed increased correspondence between replicates of the same cell type upon GC normalization ( Supplementary Fig. 5 ). Nucleosomes differ in their properties including stability, accessibility and turnover rate, and the magnitude of the nucleosomal signal detected at TSSs in a particular study reflects how well nucleosomes of each type are profiled in a specific experimental setting. For example, using different salt concentrations during chromatin isolation results in different TSS-proximal profiles [24] . Similarly, different MNase digestion levels can produce different TSS-proximal profiles, each reflecting nucleosomal signal characteristic for given experimental conditions. Therefore, to further validate our results, we assessed another target GC content (48%, which represents the average GC content of our samples), confirming that our conclusions are not limited to a specific target GC content used for normalization (see Methods). Thus, we conclude that the GC normalization effectively reduces variability present in MNase-seq data and enables comparisons of nucleosome occupancy across different cell types. Equipped with this methodology, we proceeded to identifying changes in nucleosome occupancy in pluripotent and somatic cells. Nucleosome occupancy at regulatory loci varies in cell types We began by investigating differences in nucleosome organization at gene promoters and enhancers where we hypothesized it to play a role, and then extended the analysis to the whole genome. Using normalized MNase-seq data, we initially examined nucleosome occupancy of promoters in relation to both the transcriptional status of the associated gene and the covalent-histone modifications present. Consistent with previous reports, promoters of transcriptionally active genes showed an enhanced NDR as well as pronounced phasing of nucleosomes distal to the +1 and −1 nucleosomes, while promoters of transcriptionally silent genes lacked an NDR, demonstrating instead an occupancy signal indicative of a single nucleosome located approximately at the +1 nucleosome site ( Fig. 1c ) [16] , [17] , [18] , [19] , [22] , [32] . Furthermore, an increased NDR was observed in a cell-type-specific manner for genes that were upregulated in pluripotent cells ( Supplementary Fig. 6 ). This effect was not pronounced for genes upregulated in somatic cells, suggesting that factors other than nucleosome rearrangement are responsible for silencing these genes in the pluripotent state. Pluripotent cell promoters have been extensively characterized with regard to covalent-histone marks, including histone H3 lysine 4 trimethylation (H3K4me3) and histone H3 lysine 27 trimethylation (H3K27me3), which are associated with active and silent genes, respectively. Indeed, promoters classified by H3K4me3 and H3K27me3 enrichment exhibited nucleosome occupancy profiles characteristic for corresponding transcription status ( Supplementary Fig. 7A–D ). Comparing the average nucleosome occupancy at these promoters revealed decreased and increased occupancy levels for the promoters associated with H3K4me3 and H3K27me3 enrichment, respectively ( Fig. 1d ). This observation is consistent with increased nucleosome occupancy hindering transcription on average [37] . Interestingly, despite a lack of transcriptional activity at bivalent promoters (TSSs possessing both H3K4me3 and H3K27me3) [38] , their nucleosomal profiles closely resembled those of transcriptionally active genes ( Supplementary Fig. 7E ). We note that most bivalent genes are associated with CpG islands, which may contribute to a chromatin structure that is poised for transcription activation during development [39] . Enhancers comprise another class of regulatory regions key for the pluripotent state. Here we used a recently-published set of enhancers associated with the pluripotency and reprogramming factors Oct4, Nanog and Sox2, including a subset of ‘super-enhancers’ that are unusually large and impart hyper-regulatory functions in ESCs [40] , [41] . The set comprises 8,794 enhancers, 231 of which are super-enhancers. Comparison of the nucleosome occupancy profiles around scaled ESC enhancers in somatic and pluripotent cells revealed that on an average the occupancy was lower in pluripotent cells ( Fig. 1e ), which is consistent with these regions being more accessible to regulatory proteins in pluripotent cells. The same trend was observed in human MNase-seq data for hESCs, hiPSCs and differentiated human fibroblasts ( Supplementary Fig. 8A ). For a more detailed analysis, we divided all enhancers into two groups, those having significantly lower nucleosome density (LND) or higher nucleosome density (HND) in ESCs when compared with somatic TTFs (significance based on the variability of the nucleosome density in the replicates; t -test, P -value threshold 0.05). Consistent with the results described above, the LND group comprised 353 enhancers (23 of which were super-enhancers), while the HLD group comprised only 60 enhancers (one of which was a super-enhancer). When all the TSS-proximal regions were similarly divided into LND and HND groups for comparison, the corresponding counts were 558 and 341, thus resulting in considerably less skewed group counts than those detected for enhancers. We note that more than a twofold skew in the numbers of LND and HND enhancers was also present when the comparison included all enhancers rather than being limited only to those showing statistically significant differences ( Supplementary Fig. 9A ). The expression of genes associated with enhancers from the LND and HND groups significantly differed in ESCs and somatic cells ( Fig. 1f , P =5 × 10 –3 , t -test; Supplementary Fig. 9B ), with the genes associated with LND enhancers showing higher expression than the genes associated with HND enhancers. This difference was approximately the same in magnitude as that observed for the LND and HND promoters. To further investigate how nucleosome occupancy at enhancers correlates with other features of chromatin organization, we used published data on chromatin structure and TF binding in ESCs [40] . Enhancers with LND were more likely to be bound by pluripotent TFs, exhibited active chromatin marks and were associated with stronger DNase I signal when compared with enhancers from the HND group ( Fig. 1g ). This rearrangement of the nucleosome landscape at enhancers might be a key determinant in pluripotency and differentiation, with lower nucleosome occupancy correlating with stronger enhancer activity in pluripotent cells. We conclude that the rearrangement of the nucleosome landscape at regulatory regions correlates with changes in other chromatin signatures and gene expression in a cell-type-specific manner, and that active enhancers show lower levels of nucleosome occupancy in pluripotent cells. Punctate changes at regulatory regions discern cell types We next sought to identify all RoD in the nucleosome occupancy profiles of ESCs, iPSCs and somatic cells on a genome scale, regardless of their location relative to the annotated DNA elements. Nucleosome organization is likely to undergo rearrangement as cells change fate, and visual inspection of the nucleosome occupancy profiles indeed revealed such changes ( Supplementary Fig. 10 ). However, little is known about nucleosome occupancy changes on the genomic scale, including their significance, prevalence, size and distribution, in part due to the challenges inherent in mapping these differences in mammalian cells. We applied a novel approach comparing the frequency of digestion fragments in 150-bp bins to scan the genome and generate P -value profiles, describing the significance of nucleosome occupancy differences between cell types ( Fig. 2a ). We used a false discovery rate (FDR) threshold to identify sets of significant RoDs for each pairwise cell-type comparison; we note that since this algorithm is not focused on stable nucleosome positions, it is suitable for detection of RoDs of any size (see Methods for details). To rule out the possibility that RoD detection is driven by an outlier replicate, we confirmed that the direction of change in nucleosome occupancy at RoDs is the same in all pairwise comparisons of the replicates ( Supplementary Fig. 11 ). 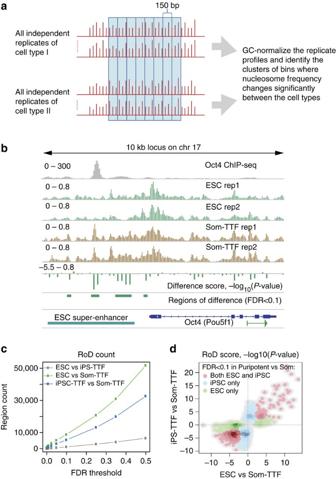Figure 2: Identification and characterization of regions of difference (RoDs) in nucleosome profiles between murine pluripotent and somatic cell types. (a) Schematic illustration of the method used for RoD identification. In short, sequenced tag frequencies in all replicates of the compared cell types (red) were binned along the genomic coordinate (blue) and the clusters of the bins where tag frequencies were significantly different were retained for further analysis (see Methods for detail). (b) Normalized nucleosome occupancy in the promoter of the Oct4 (Pou5f1) gene for two independent ESC lines and isolates of somatic TTFs. The computed difference score and identified RoDs are shown as green vertical and horizontal bars, respectively, below the occupancy tracks. The sign of the difference score indicates whether nucleosome occupancy was gained (positive score) or lost (negative score) in the ‘ESC versus somatic TTF’ comparison. The green arrow next to the gene name indicates direction of transcription. (c) Counts of the RoDs identified with different FDR thresholds (FDR=0.1 was selected to compose the representative RoD sets for the downstream analyses). (d) Correlation between difference scores of the RoDs identified in comparisons of ESCs versus somatic TTFs and iPSC-TTFs versus somatic TTFs. Only the bins that meet the FDR threshold of 0.1 at least in one comparison were taken for this analysis. Red dots represent bins that meet the selected FDR threshold in both comparisons; blue and green dots represent bins that meet the FDR threshold only in the ‘iPSC versus somatic TTF’ set or only ‘ESC versus somatic TTF’ set, respectively. We note that the sign of the score is maintained across the sets (that is, the bins that have positive (negative) scores in one pairwise cell-type comparison have the same score signs in another pairwise cell-type comparison), which is indicative of good correspondence between the loci of nucleosome occupancy variation in ESCs and iPSC-TTFs. Figure 2: Identification and characterization of regions of difference (RoDs) in nucleosome profiles between murine pluripotent and somatic cell types. ( a ) Schematic illustration of the method used for RoD identification. In short, sequenced tag frequencies in all replicates of the compared cell types (red) were binned along the genomic coordinate (blue) and the clusters of the bins where tag frequencies were significantly different were retained for further analysis (see Methods for detail). ( b ) Normalized nucleosome occupancy in the promoter of the Oct4 (Pou5f1) gene for two independent ESC lines and isolates of somatic TTFs. The computed difference score and identified RoDs are shown as green vertical and horizontal bars, respectively, below the occupancy tracks. The sign of the difference score indicates whether nucleosome occupancy was gained (positive score) or lost (negative score) in the ‘ESC versus somatic TTF’ comparison. The green arrow next to the gene name indicates direction of transcription. ( c ) Counts of the RoDs identified with different FDR thresholds (FDR=0.1 was selected to compose the representative RoD sets for the downstream analyses). ( d ) Correlation between difference scores of the RoDs identified in comparisons of ESCs versus somatic TTFs and iPSC-TTFs versus somatic TTFs. Only the bins that meet the FDR threshold of 0.1 at least in one comparison were taken for this analysis. Red dots represent bins that meet the selected FDR threshold in both comparisons; blue and green dots represent bins that meet the FDR threshold only in the ‘iPSC versus somatic TTF’ set or only ‘ESC versus somatic TTF’ set, respectively. We note that the sign of the score is maintained across the sets (that is, the bins that have positive (negative) scores in one pairwise cell-type comparison have the same score signs in another pairwise cell-type comparison), which is indicative of good correspondence between the loci of nucleosome occupancy variation in ESCs and iPSC-TTFs. Full size image Our approach is further illustrated in Fig. 2b , showing the promoter of Oct4 gene. This gene has a nucleosome occupancy pattern characteristic of an expressed gene in pluripotent cells, with an NDR at the TSS flanked by regions of high nucleosome occupancy. Somatic cells, which do not express Oct4, lack the NDR at the Oct4 TSS and show overall higher levels of nucleosome occupancy in the promoter region. Our approach was able to detect these changes and identify the RoD overlapping an Oct4 binding site important for gene upregulation in ESCs [40] . GC normalization, one of the features that distinguishes our approach from earlier algorithms [42] , facilitated the identification of RoDs by reducing variability between replicates and allowed identification of more RoDs by ~45% in the comparison of ESCs and somatic TTFs, including those at the Oct4 locus ( Supplementary Fig. 12 ). To evaluate the extent to which somatic cell reprogramming resets the chromatin structure in iPSCs, we compared the numbers of RoDs identified between pluripotent and somatic cell types with those detected between ESCs and iPSCs. As the number of detected RoDs is a function of the selected significance threshold, we analyzed RoD counts for a series of FDR thresholds. We consistently identified more RoDs in pluripotent versus somatic cell comparisons than comparisons of two independent pluripotent cell lines ( Fig. 2c ). For instance, at FDR=0.1, we identified over 8,000 RoDs when ESCs were compared with somatic TTFs, and over 5,000 RoDs when iPSCs were compared with somatic TTFs. For the ESCs and iPSC comparison, 1,041 RoDs were identified, which is five to eightfold lower than the number of RoDs identified in any pluripotent versus somatic cell comparison. We note that the transcriptional profiles of ESCs and iPSCs were very similar ( Supplementary Fig. 1F ), with <50 genes demonstrating significant changes in expression (see Methods for details on calling differentially expressed genes), which is consistent with the low number of RoDs detected when comparing these cell types. iPSCs could more closely resemble their cell of origin rather than ESCs with regard to nucleosome placing. However, based on previous work, ESCs and iPSCs are functionally equivalent and very similar at the molecular level (reviewed in ref. 43 ), and thus one would anticipate a high degree of similarity between iPSCs and ESCs in nucleosomal occupancy profiles. Indeed, the differences in nucleosome organization observed in the comparisons of somatic cells to ESCs correlate with the differences detected in comparisons with iPSCs ( Fig. 2d ). For instance, all the regions determined for a selected FDR threshold in ESCs exhibit the same directional change in the iPSC comparison, and vice versa (green and blue dots in Fig. 2d ). These observations were further confirmed in hESC, hiPSC and human fibroblast comparisons ( Supplementary Fig. 4C,D ). We also examined two basic characteristics of RoDs: their size distributions and the direction of nucleosome occupancy change. Surprisingly, while nucleosomes with altered occupancy might cluster, a vast majority of RoDs appeared to be 150 bp in size (>95% in both the mouse and human data). A small percentage (<1%) of RoDs were several kilobases in length, but no regions >0 kb were observed ( Supplementary Fig. 13 ). We note that the resolution of our approach as well as the smallest RoD size that can be reported is 150 bp, which is the size of the bins used for this analysis. Therefore, we cannot distinguish between changes occurring on mononucleosomal versus subnucleosomal scales. Our technique, however, would detect changes occurring on larger scales as those spanning multiple adjacent bins. Low count of RoDs exceeding 150 bp allows us to conclude that such large-scale changes in nucleosome occupancy are infrequent, suggesting tight control of chromatin structure at the level of single nucleosomes. When directionality of the occupancy change was considered, the majority of the RoDs identified between pluripotent and somatic cells showed an increase in nucleosome signal in the differentiated cells ( Fig. 3a , see Supplementary Fig. 4E for human data). This supports the hypothesis that pluripotent cells have relatively open chromatin, as one criterion for open chromatin would be lower nucleosome occupancy. The RoDs identified between ESCs and iPSCs showed little bias in nucleosome occupancy change direction, suggesting the absence of a dominant trend distinguishing the chromatin structure in these cells. 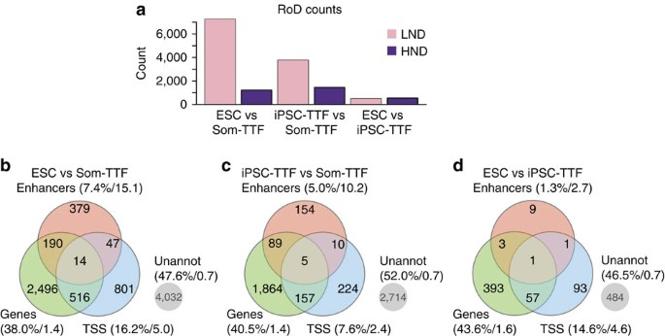Figure 3: Occurrences of the regions of difference (RoDs) identified in pairwise comparisons of mouse cell types. (a) Comparison of the counts of RoDs with lower (pink) and higher (purple) levels of nucleosome occupancy in the pluripotent cell types relative to somatic TTFs (first two bar groups) and in ESCs relative to iPSCs (last bar group). (b–d) Occurrences of the identified RoDs in the different regions of the genome for pairwise comparisons of ESCs versus somatic TTFs (b) iPS-TTFs versus somatic TTFs (c), and ESCs versus iPSC-TTFs (d). Genes are defined according to USCS annotation for mm9 genome, TSS-proximal regions comprise ±2 kb around gene starts, and ESC enhancer coordinates were taken from a recent publication40. The numbers inside the circles represent counts of RoDs in corresponding regions. The numbers next to the region name represent the percentage of the RoD occurrences in this region to the total RoD count and the enrichment of this percentage over the expected value based on the region size in the genome. We note that the evaluated regions can overlap and therefore the sum of the percentages is not equal to 100%. This figure only includes RoDs meeting a FDR=0.1. Figure 3: Occurrences of the regions of difference (RoDs) identified in pairwise comparisons of mouse cell types. ( a ) Comparison of the counts of RoDs with lower (pink) and higher (purple) levels of nucleosome occupancy in the pluripotent cell types relative to somatic TTFs (first two bar groups) and in ESCs relative to iPSCs (last bar group). ( b – d ) Occurrences of the identified RoDs in the different regions of the genome for pairwise comparisons of ESCs versus somatic TTFs ( b ) iPS-TTFs versus somatic TTFs ( c ), and ESCs versus iPSC-TTFs ( d ). Genes are defined according to USCS annotation for mm9 genome, TSS-proximal regions comprise ±2 kb around gene starts, and ESC enhancer coordinates were taken from a recent publication [40] . The numbers inside the circles represent counts of RoDs in corresponding regions. The numbers next to the region name represent the percentage of the RoD occurrences in this region to the total RoD count and the enrichment of this percentage over the expected value based on the region size in the genome. We note that the evaluated regions can overlap and therefore the sum of the percentages is not equal to 100%. This figure only includes RoDs meeting a FDR=0.1. Full size image Thus our analysis revealed mostly punctate differences in nucleosome occupancy between pluripotent and somatic cells. These loci are predominantly associated with lower nucleosome occupancy in pluripotent cells. Overall, ESCs and iPSCs display a high degree of similarity in nucleosomal signal, providing evidence that somatic cell reprogramming resets nucleosome positioning to a pluripotent state [44] . We next sought to more fully characterized RoD locations, as these regions are likely regulatory sites involved in pluripotency and reprogramming. RoDs are enriched at regulatory regions active in ESCs Our analysis showed that ~40% of RoDs are at gene regions annotated in the mouse genome ( Fig. 3b–d , see also Fig. 4a , Supplementary Fig. 8B ), which is significantly more than expected for a randomized distribution ( P =10 −12 , see Methods for details on significance estimation). Around genes, TSS-proximal regions are specifically enriched in RoDs ( Fig. 4c , blue line), including the promoters of genes associated with pluripotency and transcription activation (as exemplified by Oct4 in Fig. 2b ). Indeed, in pluripotent versus somatic cell comparisons, between 7 and 16% of RoDs occur at TSSs, and these are enriched 2.4 to 5 fold over the genome average ( Fig. 3b,c ). In addition to genes and their promoters, pluripotency-associated enhancers exhibited significant enrichment in RoDs ( Fig. 4c , orange line, and Supplementary Fig. 8C ). To our surprise, enhancers demonstrated differences with the same or greater magnitude as TSSs. In pluripotent versus somatic cell comparisons, between 5 and 7.4% of RoDs occurred at ESC-defined enhancers, which corresponds to a 10- to 15-fold enrichment over the genome-wide occurrence of these enhancers ( Fig. 3b,c ). ‘Super-enhancers’—large enhancer regions associated with a high density of regulatory protein binding [40] —showed even stronger enrichment in RoDs ( Fig. 4c , red line). As an additional validation of this result, we identified RoDs between ESCs and another somatic cell type, mouse liver. This set of RoDs was also skewed towards LND enhancers in ESCs and showed enrichment at TSSs and ESC enhancers ( Supplementary Fig. 14 ), confirming that these effects are not specific to the somatic cell type to which ESCs are compared. 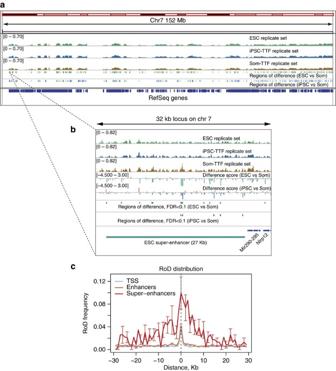Figure 4: Distribution of the regions of difference (RoDs) detected in nucleosome occupancy profiles relative to annotated regions in the mouse genome. (a) Chromosome wide snapshot of the normalized nucleosome occupancy and RoD occurrence. (b) Nucleosome occupancy at one of the super-enhancers identified in Whyteet al.40shown as an example of multiple RoDs present in this class of enhancers. (c) The RoD frequencies in the regions encompassing TSSs and enhancers identified in ESCs40. The 95% confidence intervals are shown with the vertical arrows. The confidence intervals were estimated based on the variability of the frequency values in individual profiles used for averaging. Figure 4: Distribution of the regions of difference (RoDs) detected in nucleosome occupancy profiles relative to annotated regions in the mouse genome. ( a ) Chromosome wide snapshot of the normalized nucleosome occupancy and RoD occurrence. ( b ) Nucleosome occupancy at one of the super-enhancers identified in Whyte et al . [40] shown as an example of multiple RoDs present in this class of enhancers. ( c ) The RoD frequencies in the regions encompassing TSSs and enhancers identified in ESCs [40] . The 95% confidence intervals are shown with the vertical arrows. The confidence intervals were estimated based on the variability of the frequency values in individual profiles used for averaging. Full size image To further quantify the overlap between RoDs and these regulatory regions, we computed the percentage of enhancers and TSSs harbouring RoDs. We note that actual values of such an overlap would depend on the sequencing depth achieved in a particular study (that is, statistical power to identify RoDs and enhancers) and the significance threshold used to call RoDs. Under the threshold used in this study, we found that 7% of ‘regular’ enhancers and 39% of super-enhancers bear at least one RoD, which represents a significant overlap as compared with the expected value for randomized RoD distributions ( P =10 −11 , see Methods). A similar fraction of TSS-proximal regions (6%) harbour RoDs, which reinforces the importance of chromatin structure and its regulation at enhancers in pluripotent and somatic cells. While most enhancers harbour only one or no RoDs, super-enhancers are often associated with multiple RoDs. An example of such a super-enhancer is given in Fig. 4b , where up to nine RoDs, all from the LND group, can be detected. RoDs are enriched in binding motifs of reprogramming TFs Given that the detected RoDs are small in size (~150 bp) and enriched at regulatory sites, one could hypothesize that they are associated with regulatory protein binding that displaces a single nucleosome. For instance, regions associated with binding of TF involved in cell differentiation were reported to have lower nucleosome occupancy in the corresponding somatic cell type [21] . Here we focused on the regions with lower nucleosome occupancy in pluripotent cells (LND RoDs) and analyzed them for the presence of sequence motifs to identify potential regulatory factors. We found that mouse LND RoDs identified in comparison of ESCs and somatic cells were enriched in motifs of TFs associated with reprogramming and pluripotency, including Klf4, c-Myc, Oct4 and Stat3 ( Fig. 5a , Supplementary Fig. 15 ). As Oct4 and Sox2 act as heterodimers in pluripotent cells [45] , [46] , [47] , we conclude that our analysis identifies potential sites of functional binding for all four Yamanaka reprogramming factors. The Stat3 motif is also highly enriched in these RoDs, and Stat3 is required and sufficient for the self-renewal of mouse ESCs [48] . Performing a de novo motif search with a random set of genomic sequences mimicking the RoD set did not reveal motifs for the Yamanaka factors (with the selected significance threshold of E -value=10 −5 ). We note that many of the factors associated with the motifs identified within the RoDs also bind enhancers in pluripotent cells and, furthermore, their binding is often used to define enhancers in pluripotent cells [40] , [47] . 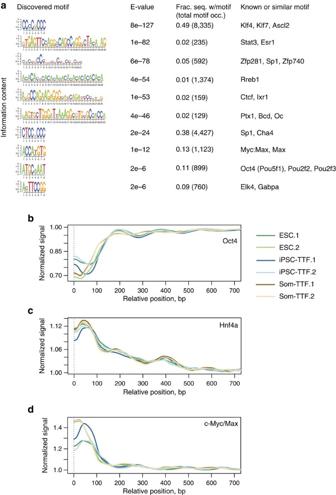Figure 5: Relation between local nucleosome organization and the presence of TF binding motifs. (a) Sequence motifs found inde novoenrichment analysis of the RoDs associated with lower nucleosome occupancy levels in ESCs as compared with somatic TTF cells. CorrespondingE-values are indicated for each motif as well as the fractions of the test sequences with the motifs and total occurrences of the motifs in the sequence set, computed for 85% identity threshold. The last column lists the TFs associated with similar motifs. Motifs with no known associated protein and those <8 bp in length are not shown (seeSupplementary Fig. 15for a complete list of the identified motifs). (b–d) Distribution of nucleosome occupancy around the motifs of selected TFs, (b) Oct4, (c) Hnf4a and (d) c-Myc/Max. The occupancy was averaged over all motifs identified in the mouse genome with the selected FDR threshold and the plot was symmetrized relative to the motif center. Figure 5: Relation between local nucleosome organization and the presence of TF binding motifs. ( a ) Sequence motifs found in de novo enrichment analysis of the RoDs associated with lower nucleosome occupancy levels in ESCs as compared with somatic TTF cells. Corresponding E -values are indicated for each motif as well as the fractions of the test sequences with the motifs and total occurrences of the motifs in the sequence set, computed for 85% identity threshold. The last column lists the TFs associated with similar motifs. Motifs with no known associated protein and those <8 bp in length are not shown (see Supplementary Fig. 15 for a complete list of the identified motifs). ( b – d ) Distribution of nucleosome occupancy around the motifs of selected TFs, ( b ) Oct4, ( c ) Hnf4a and ( d ) c-Myc/Max. The occupancy was averaged over all motifs identified in the mouse genome with the selected FDR threshold and the plot was symmetrized relative to the motif center. Full size image Protein binding was previously shown to order nucleosomes on a scale larger than the 150 bp observed for most of the RoDs in our analysis [18] , [49] , [50] . We therefore examined how TF binding may affect nucleosome occupancy beyond the RoD boundaries in different cell types. To this end, we compared the nucleosome profiles around TF binding motifs in each cell type. Our results show that such TF-proximal nucleosome profiles exhibit unique properties depending on the TF considered. For the Oct4 motif, we observed clear nucleosome phasing emanating away from the Oct4 binding site in pluripotent cells but not in somatic TTFs, which lack Oct4 expression ( Fig. 5b ). Conversely, for a TF specific for differentiated cells, Hnf4a, we observed phasing in somatic but not in pluripotent cells ( Fig. 5c ). For c-Myc/Max (a TF that is expressed in ESCs, iPSCs and somatic TTFs), we observed nucleosome phasing in all samples ( Fig. 5d ). Interestingly, there is a shift in phasing with c-Myc/Max in pluripotent and somatic cells, which may indicate preferential binding of this TF to different genomic regions in these cell types. Together, these data support that local changes in nucleosome occupancy are formed around TF binding sites and suggest that the cell-specific TF expression and binding helps to establish the unique chromatin context for a given cell type [26] , [51] , [52] . To further validate that RoDs reflect TF binding sites, we investigated the enrichment of ChIP-Seq signal at these loci, using data on pluripotency-associated TF binding from an independent study [40] . Our results revealed several-fold enrichment in Oct4, Sox2 and Nanog signal at LND RoDs, while no such enrichment was detected for HND RoDs ( Fig. 6a–d ). In addition, the profile of H3K4me3, also based on ESC data, showed a clear drop at the center of LND RoDs, which is consistent with nucleosome depletion. These findings highlight a possible role for TF binding in the rearrangement of nucleosomal landscape and suggest that different factors are responsible for the emergence of LND and HND RoDs. 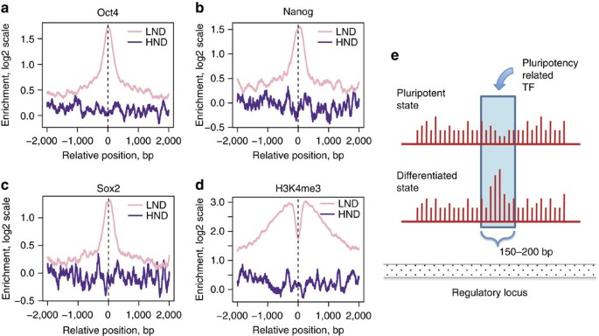Figure 6: TF binding at the sites of nucleosome rearrangement. Enrichment profiles (ChIP over WCE input) computed in the RoD proximal regions for (a) Oct4, (b) Nanog, (c) Sox2 and (d) H3K4me3 mark. Two classes of RoDs are considered separately: LND (light pink) and HND (purple). (e) Schematic summary of the observations reported in this paper. While nucleosome occupancy profiles (red vertical bars) remain similar between the pluripotent and differentiated states, there are punctate regions of difference (marked by the light blue rectangle) characterized by lower nucleosome occupancy in the pluripotent state. Majority of these regions do not exceed the size of a single nucleosome. They are enriched in binding motifs of pluripotency-related TFs and occur within regulatory regions, such as gene promoters and enhancers. Figure 6: TF binding at the sites of nucleosome rearrangement. Enrichment profiles (ChIP over WCE input) computed in the RoD proximal regions for ( a ) Oct4, ( b ) Nanog, ( c ) Sox2 and ( d ) H3K4me3 mark. Two classes of RoDs are considered separately: LND (light pink) and HND (purple). ( e ) Schematic summary of the observations reported in this paper. While nucleosome occupancy profiles (red vertical bars) remain similar between the pluripotent and differentiated states, there are punctate regions of difference (marked by the light blue rectangle) characterized by lower nucleosome occupancy in the pluripotent state. Majority of these regions do not exceed the size of a single nucleosome. They are enriched in binding motifs of pluripotency-related TFs and occur within regulatory regions, such as gene promoters and enhancers. Full size image Overall, our results revealed that the differences in nucleosome occupancy profiles in pluripotent and somatic cells mostly appear as punctate changes at individual loci. These differences tend to cluster at regulatory regions that control gene expression, including promoters and enhancers of developmentally regulated genes, indicating their functional importance for determining the regulation of cell status. We conclude that these are not wholesale changes in nucleosome positioning between pluripotent and somatic lineages, but rather specific changes whose location implies a key role in the transition between cell states. The objective of this study was to determine the nature of changes that occur in nucleosome occupancy profiles upon transition between pluripotent and somatic cells. To address this question, we used MNase digestion assays as the primary tool. We note that while the extent to which MNase-associated bias affects the determination of nucleosome positioning is still debated [33] , [53] , the design of our study, which involves an additional step for bias correction and focuses on pairwise comparison of the occupancy profiles, minimizes the possibility of artifacts. One can expect that a dramatic change in cell identity, such as that occurring during somatic cell reprogramming or differentiation of pluripotent cells, would be accompanied by large-scale changes in primary chromatin structure. To our surprise, we detected only a handful of RoDs larger than 1 kb in size. At the same time, we observed a number of important features in the re-organization of nucleosomal landscapes associated with pluripotency. Our main conclusions are that changes in nucleosome occupancy largely do not exceed mononucleosomal size, co-localize with binding sites of pluripotency and reprogramming associated proteins, generally have reduced levels of nucleosome occupancy in pluripotent cells, and are enriched at enhancers, promoters and within genes ( Figs 3b–d and 6e ). Comparisons of different classes of regulatory regions revealed that RoDs at enhancers and especially at super-enhancers are at least as prevalent as those at TSSs, underscoring the importance of these regions in determining cell state [40] , [41] , [54] . Another central conclusion is that fully reprogrammed and characterized iPSCs [28] , [55] demonstrate nucleosome occupancy patterns similar to those in blastocyst-derived ESCs, with eightfold fewer RoDs detected between ESCs and iPSCs than between ESCs and somatic TTFs. Importantly, the nucleosome configuration at enhancers in iPSCs is similar to that in ESCs, while it is considerably different from that in fibroblasts. In addition, the RoDs identified between pluripotent and somatic cells contained binding motifs for the Yamanaka reprogramming factors as well as other key pluripotency factors, suggesting that the nucleosome occupancy changes overlap with the regulatory regions that are important for cell identity. Chromatin structure in general, and nucleosome occupancy in particular, could represent an additional and fundamental level of epigenetic memory that must be reset for proper somatic cell reprogramming [54] , [56] . Our analysis supports, from a distinct angle, the previously-reported observation that pluripotent cells have more ‘open’ chromatin compared with somatic cells. ChIP-seq on H3K9me3 and H3K27me3 suggested that these heterochromatic marks cover over three times more of the genome in differentiated cells when compared with ESCs [57] . In addition, the nuclei of pluripotent cells have macroscopic characteristics of less-condensed chromatin, histone turnover appears more dynamic in pluripotent cells, and regulatory regions show enrichment in histone variants and covalent modifications that are characteristic of open chromatin [4] , [58] . Here we observe that a majority of the detected RoDs are associated with lower nucleosome occupancy in pluripotent cells when compared with somatic cells. The lower nucleosome occupancy in pluripotent cells correlates with function, since it is predominantly observed at active chromatin regions, including ESC-specific enhancers and promoters of genes upregulated in ESCs and iPSCs. We conclude that the more permissive chromatin configuration in pluripotent cells is enabled not only through reduction of the heterochromatic regions but also through local changes in the nucleosomal landscapes of euchromatic regions. While most of RoDs do not appear to exceed the size of a single nucleosome, we note that protein binding may induce larger-scale rearrangement of chromatin, such as the increased nucleosome phasing observed in Fig. 5b–d . However, deeper sequencing and a larger number of replicates would be required to identify a ‘complete’ set of RoDs, which would include such changes at individual loci. In combination with protein-binding motif information, our current approach can be used for simultaneous identification of nucleosome rearrangement and differential binding for a range of TFs in one assay, when such data are available. This approach could be further enhanced by analyzing the digested fragments of subnucleosomal sizes and/or by using multiple levels of digestion for the same sample to preferentially profile genomic loci of different accessibility [30] , [59] . Such a comprehensive approach would help us better understand how changes in chromatin organization translate into changes in gene expression and cell identity. Experimental procedures Cell culture Mouse ESCs and iPSCs were maintained on mouse embryonic fibroblast feeder layers (Specialty Media) in DMEM containing 15% heat-inactivated foetal bovine serum (Hyclone) supplemented with 1,000 U ml −1 leukaemia Inhibitory Factor (Chemicon). The following mouse cell lines were used in these studies: A5 ESCs (ESC.1), A6 ESCs (ESC.2), A4 iPSCs (iPS.TTF.1) and A5 iPSCs (iPS.TTF.2). All isogenic lines were created from mice containing the stable integration of doxycycline-inducible reprogramming factors (Oct4, Sox2, Klf4 and c-Myc). All experiments were initiated with cell lines between passage 15 and 22. Primary TTFs and liver were obtained as secondary derivates from B6/129 neonatal mice aged between 7 and 14 days postpartum. These mice and cell lines have been functionally characterized and were previously reported [25] . Human ESCs and iPSCs were maintained on Geltrex (Life Technologies) in mTeSR1 (Stem Cell Technologies). H1-OGN ESCs [60] and iPSCs [28] were functionally characterized previously [28] , [60] . These cells exhibited the expected in vitro molecular and functional properties of human pluripotent cells in our hands, but showed low to no OCT4-GFP reporter expression. Experiments were carried out with H1-OGN ESCs between passage 76 and 77 and iPSCs between passage 14 and 17. Differentiated fibroblasts were made from H1-OGN ESCs and were used between passages 7 and 14. Chromatin digestion with MNase Each murine cell type was expanded to ~3 × 10 7 cells and pretreated with mild detergents (0.2% Tween-20 and 0.2% Triton X-100) for 5 min followed by a 1.1% formaldehyde treatment for 10 min to preserve chromatin structure. Nuclei were then prepared from the cross-linked cells and the chromatin treated with three MNase concentrations for 15 min at room temperature (RT). A range of digestion conditions was employed to sample both hyper- and hypo-accessible chromatin regions to MNase digestion. Cross-links were then reversed for 16 h at 55 °C along with proteinase K digestion and DNA harvested via phenol–chloroform. Samples were then run on 1% agarose gels and the resulting mononucleosomal DNA fragments (~150 bp) were gel purified, pooled and prepared for sequencing on an Illumina HiSeq instrument. Human cells were expanded to ~1 × 10 8 cells and cross-linked with 1.1% formaldehyde for 10 min at RT. Nuclei were isolated and treated with a range of four MNase concentrations for 15 min at RT. Cross-link reversal was performed at 65 °C for at least 16 h followed by an RNase and subsequent proteinase K digestion. DNA was purified by phenol–chloroform extraction. Ampure SPRI beads (Beckman Coulter) were used in a double size selection with ratios of 0.7 × and 1.7 × to obtain a range of fragment sizes from ~100 to 1,000 bp. The resulting sample contains a majority of mononucleosomal fragments with some smaller and di-nucleosome-sized fragments with high reproducibility. The resulting fragments from each MNase concentration in the range were prepared individually for barcoded sequencing on an Illumina HiSeq instrument. Mapped read from all concentration were subsequently pooled for analysis. Illumina HiSeq library preparation and sequencing Mononucleosome DNA (1 μg) was used for library preparation, with limited number of PCR amplification rounds [61] , and genomic alignments of paired-end 50 bp reads were performed using Bowtie [62] followed by further tag processing and filtering with the SPP workflow [28] . All alignments and annotations used the mouse genome assembly mm9 and the human genome assembly hg19. Transcriptional profiling RNA samples from each cell line were purified using TRIZOL (Invitrogen), and double-stranded complementary DNA (cDNA) was generated using the SuperScript double-stranded cDNA kit (Invitrogen). Samples were then submitted to Roche NimbleGen for subsequent hybridization and downstream processing using the NimbleGen 12 × 135 k mouse gene expression array platform, which assays 44,170 target genes with three separate 60mer probes per transcript. Biological replicates were performed for all cell lines. Bioinformatic and statistical data analysis Sequencing data preprocessing and initial analysis See Supplementary Table 1 for the number of tags and the insert size for each sample. Sequenced 50-bp paired-end tags were mapped to the mouse (mm9) or human genome (hg19) for the corresponding cell types using the Bowtie aligner v. 0.12.7 (ref. 62) [62] . Only uniquely mapped tags with no more than two mismatches in the first 28 bp of the tag were retained. Genomic positions with the number of mapped tags above the significance threshold of z -score=7 were identified as anomalous, and the tags mapped to such positions were discarded. The coordinates of the genes were taken according to the annotations for mm9 and hg19 versions of the mouse and human genomes, respectively. The gene proximal profiles were calculated and plotted as described previously [29] , [63] . GC-content normalization The GC-correction procedure applied in this study is illustrated in Supplementary Fig. 3 . The correction coefficient for each read was computed in such a way that the resulting genome-wide distributions of GC content become similar to the target GC-content distribution (Gaussian distribution with mean GC=50 and 48% and variance=7.5%). Specifically, all reads were stratified according to the GC content of the regions ±100 bp around mapping location of the pair-end read centres and the correction coefficients were computed as ratios of the histograms corresponding to experimental and theoretical GC-content distributions with 1% GC-content step. The coefficients were applied to the tag frequencies at each genomic position with non-zero tag counts. For the purpose of RoD identification, the corrected tag frequencies were rounded to the closest integer. The value of GC=50% was used to obtain main results in the study, and GC=48% was used for validation purposes to confirm that the same trends can be observed in downstream analyses with other target GC-content values ( Supplementary Fig. 16 ). Detecting RoD in nucleosome occupancy P -values of the differences were estimated for the frequency of reads summarized within 150-bp non-overlapping bins. The P -value calculation was based on the negative binomial distribution, with variance and mean estimated based on the replicate profiles produced for each cell type, as implemented in the R package DESeq [64] . Default parameters of DESeq were used for computations. To account for local context of nucleosome occupancy, the estimation of significance of the nucleosome occupancy changes within bins was performed independently in 25 kb segments with a 12.5 kb step, hence generating two significance values for each bin. The more conservative estimate was retained for further analysis. The bins exhibiting significant changes in tag frequency between the samples separated by >100 bp were merged to form RoD. Coordinates of the identified RoDs are provided as Supplementary Files . Estimation of statistical significance Significance estimations were performed using R ( http://www.r-project.org ). Abundances of RoDs in genomic regions were compared with the corresponding values obtained for the randomized RoD distributions in mappable regions of the genome using non-parametric Wilcoxon test (as implemented in the function ‘wilcox.test’ from the package ‘stats’). Only the regions of the genome that had non-zero tag counts were used in randomization (at least 1,000 randomizations were performed in each case). Gene expression data processing Gene expression data for mouse cells were generated using the NimbleGen expression micorarrays (Roche NimbleGen, Inc., Madison, WI). Microarray data provided by NimbleGen were background-corrected and normalized between the arrays using the Robust Multichip Average approach. Fold-change and statistical significance were estimated for the expression values of each gene based on the data for individual replicates within each replicate set. The genes with at least twofold change in expression and meeting a P -value threshold of 0.05 were identified as differentially expressed. Motif analysis Motif analysis was performed using web-base service MEME-ChIP [65] . Motifs that are at least 6 bp in length identified with an E -value threshold of 10 −5 were reported. Both palindromic and non-palindromic motifs were allowed. The motifs found in the test sequences were matched against JASPAR (CORE-2009) or UniPROBE (mouse) databases to identify similarity with known protein motifs using tools implemented in MEME-ChIP with default parameters. Calculation of motif occurrences in test sequences and sequence logo generation were performed using the Bioconductor packages Biostrings and seqLogo, respectively ( http://www.bioconductor.org ). How to cite this article: West, J. A. et al . Nucleosomal occupancy changes locally over key regulatory regions during cell differentiation and reprogramming. Nat. Commun. 5:4719 doi: 10.1038/ncomms5719 (2014). Accession codes: All data sets are available in the NIH GEO database under accession code GSE59064 .